Self-assembly of DNA nanotubes with controllable diameters The synthesis of DNA nanotubes is an important area in nanobiotechnology. Different methods to assemble DNA nanotubes have been reported, and control over the width of the nanotubes has been achieved by programmed subunits of DNA tiles. Here we report the self-assembly of DNA nanotubes with controllable diameters. The DNA nanotubes are formed by the self-organization of single-stranded DNAs, exhibiting appropriate complementarities that yield hexagon (small or large) and tetragon geometries. In the presence of rolling circle amplification strands, that exhibit partial complementarities to the edges of the hexagon- or tetragon-building units, non-bundled DNA nanotubes of controlled diameters can be formed. The formation of the DNA tubes, and the control over the diameters of the generated nanotubes, are attributed to the thermodynamically favoured unidirectional growth of the sheets of the respective subunits, followed subjected to the folding of sheets by elastic-energy penalties that are compensated by favoured binding energies. The synthesis of DNA nanotubes attracts research efforts because of the possible applications of these nanostructures as containers for the transport and release of nano-cargos [1] , [2] , the use of the nanotubes as templates for the shape- and size-controlled growth of nano-objects [3] , and the incorporation of the nanotubes as functional elements in nano-devices [4] . The synthesis of programmed one-, two- and three-dimensional DNA nanostructures is a rapidly developing research topic [5] , [6] , [7] , and the resulting DNA assemblies were used as templates for the precise positioning of nanoparticles [8] , [9] , [10] and proteins [11] , [12] , [13] , [14] . Different methods have been used to assemble DNA nanotubes, and these include the self-assembly of triple-cross-over tiles [15] , the closure of two-dimensional tiles or circular arrays by complementary hybridization [16] , the self-assembly of a single DNA tile with internal complementarity [17] , or covalent bonds [18] . Also, the synthesis of geometrically defined single-stranded DNA, rigidified with organic vertices that are longitudinally assembled into nanotubules [19] , the synthesis of DNA nanotubes of predetermined lengths [20] and the templated synthesis of nanotubes have been reported [21] . The control over the width of the DNA nanotubes can be achieved through the self-assembly of a controlled number of triple-cross-over tiles and helix-arched motifs [22] , by programming the circumferences of the tubes by the complementarity of domains in single-stranded DNA [23] , and by the nano-engineered closure of origami nanotubes by appropriate 'staple' units [24] . The development of new methodologies for controlling the diameter of DNA nanotubes is important for further advancing DNA nanotechnology. Here we report a method for the high throughput synthesis of single, non-branched DNA nanotubes, where control over the diameter of the nanotubes is achieved. Specifically, we introduce a method to dictate the unidirectional growth of a sheet of DNA subunits using a rolling circle amplification (RCA) product as a template, and control its folding through the energetics involved with the displacement of the RCA template. Furthermore, we attempt to provide a simple model that accounts for the formation of the single nanotubes with controllable diameters. Bundled nanotubes assembled by hexagon subunits The single-stranded nucleic acid ( 1 ; Fig. 1 ) consists of 100 bases. The sequence is designed in such a way that domain I and VII are complementary to the sequence IV, the sequence II is complementary to region V and the sequence III is complementary to domain VI. The 3′ end of domain VII includes a toehold nucleic acid VIII. 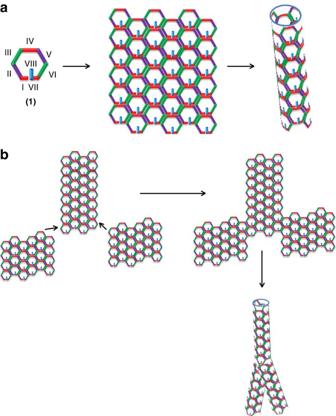Figure 1: Schematic formation of the DNA nanotubes. (a) Self-assembly of a single-stranded nucleic acid 'hexagon' subunit (1) into a 'graphene'-type sheet and its folding to a DNA nanotube. Domains I and VII are complementary to domain IV, domain II is complementary to domain V and domain III is complementary to domain VI. Domain VIII acts as a toehold for the further attachment of nanoparticles. (b) The self-assembly of nucleic acid sheets consisting of 'hexagon' subunits into bundles of DNA nanotubes. The complementarity features of the single-stranded nucleic acid ( 1 ), yield a hexagon-type structure that may inter-hybridize with other hexagon-type strands to form two-dimensional 'graphene-like' sheets that could wrap into three-dimensional tubes, as schematically outlined in Figure 1 . Figure 1: Schematic formation of the DNA nanotubes. ( a ) Self-assembly of a single-stranded nucleic acid 'hexagon' subunit ( 1 ) into a 'graphene'-type sheet and its folding to a DNA nanotube. Domains I and VII are complementary to domain IV, domain II is complementary to domain V and domain III is complementary to domain VI. Domain VIII acts as a toehold for the further attachment of nanoparticles. ( b ) The self-assembly of nucleic acid sheets consisting of 'hexagon' subunits into bundles of DNA nanotubes. 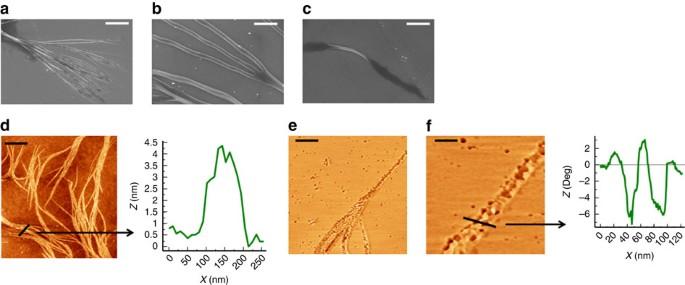Figure 2: HR-SEM and AFM images of nanostructures generated by the self-assembly of the nucleic acid subunit (1). (a) A collection of DNA nanotubes bundle merging from a central DNA tube (scale bar, 5 μm). (b) A 'zoom-in' image of DNA bundles merging from a central DNA tube (scale bar, 500 nm). (c) An image of a DNA nanotube terminated at its ends with unfolded DNA sheets of 'hexagon' units (scale bar, 700 nm). (d) AFM image of the DNA nanotubes bundles generated upon the self-assembly of the1, 'hexagon'-type subunit (scale bar, 900 nm). (e) Phase AFM image of a DNA nanotubes bundle generated upon the self-assembly of1. The dark dots in the nanostructure correspond to the 'hexagon' holes comprising the tubes (scale bar, 300 nm). (f) Zoom-in of the phase AFM image of the nanotubes and the respective cross-section analysis. Note that after tip diameter deconvolution the width of the 'holes' corresponds to∼10 nm consistent with the geometrical dimension of the respective nucleic acid 'hexagon' subunit (scale bar, 100 nm). Full size image The high-resolution (HR)-scanning electron microscopy (SEM) and atomic force microscopy (AFM) images of the resulting nanostructures are shown in Figure 2 . The typical self-assembled nanostructures consist of bundles of tubes of revealing variable diameters ( Fig. 2a ). The resulting tubes are often of a large diameter of ca 200 nm that branches into tubes of smaller diameters, ca 60 nm ( Fig. 2b ). Among the generated tubes one may trace incompletely folded nanotubes. For example, Figure 2c shows a nanostructure whose central part is folded into a tube, while its two ends exist as unfolded two-dimensional arrays. Such composite DNA tubes that include incompletely wrapped structures are often detected in the images. Very similar conclusions are derived from AFM images. The most frequent nanostructures (>90%) are composed of DNA bundles of variable diameters ( Fig. 2d ). Figure 2e,f shows the phase images of one of the bundles. The cross-section analysis of the 'holes' in the tube is shown in Figure 2f . Taking into account the tip dimensions of the AFM tip, the diameter of the holes is ca 10 nm consistent with the dimensions of the 90-base hexagons that are inter-moleculary hybridized. The formation of the hexagon-based nanotube bundles may be attributed to the random growth of the hexagon sheet, or the random inter-hybridization of hexagon sheet subunits, followed by their wrapping into nanotubes, as schematically depicted in Figure 1b . Figure 2: HR-SEM and AFM images of nanostructures generated by the self-assembly of the nucleic acid subunit ( 1 ). ( a ) A collection of DNA nanotubes bundle merging from a central DNA tube (scale bar, 5 μm). ( b ) A 'zoom-in' image of DNA bundles merging from a central DNA tube (scale bar, 500 nm). ( c ) An image of a DNA nanotube terminated at its ends with unfolded DNA sheets of 'hexagon' units (scale bar, 700 nm). ( d ) AFM image of the DNA nanotubes bundles generated upon the self-assembly of the 1 , 'hexagon'-type subunit (scale bar, 900 nm). ( e ) Phase AFM image of a DNA nanotubes bundle generated upon the self-assembly of 1 . The dark dots in the nanostructure correspond to the 'hexagon' holes comprising the tubes (scale bar, 300 nm). ( f ) Zoom-in of the phase AFM image of the nanotubes and the respective cross-section analysis. Note that after tip diameter deconvolution the width of the 'holes' corresponds to ∼ 10 nm consistent with the geometrical dimension of the respective nucleic acid 'hexagon' subunit (scale bar, 100 nm). Full size image Single-DNA nanotubes formed by hexagon or tetragon subunits Major challenges in the fabrication of DNA nanotubes involve, however, the development of methods to synthesize single, non-bundled, DNA nanotubes, and particularly, the introduction of means to control the diameter of the tubes. Towards this goal we decided to dictate the growth of the hexagon sheet by means of pre-synthesized RCA single-strand chain that is complementary to one edge of the hexagon sheet ( Fig. 3a ). The wrapping of the sheet with the concomitant displacement of the RCA blocker ( 7 ) is, then, anticipated to yield the DNA nanotube. Surprisingly, only single, non-bundled, DNA nanotubes are formed. 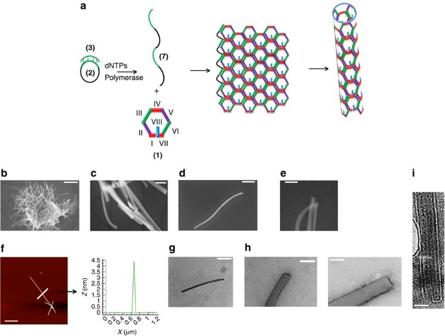Figure 3: Self-assembly and images of single-DNA nanotubes comprised of hexagon subunits. (a) Schematic formation of a single-DNA nanotube through the self-assembly of the nucleic acid 'hexagon' subunit (1), in the presence of an RCA template (7) that is partially complementary to the hexagon subunits. (b–e) HR-SEM images of the resulting single-DNA nanotubes: (b) a collection of numerous nanotubes (scale bar, 2 μm). (c) Zoom-in image of the resulting nanotubes (scale bar, 150 nm). (d) A representative image of a single micrometre-long DNA nanotube (scale bar, 500 nm). (e) Zoom-in image of the edge of a single nanotube, exhibiting the cavity of the tube (scale bar, 300 nm). (f) AFM height image of a collection of separated DNA nanotubes (scale bar, 1.7 μm). (g–i) HR-TEM images of the DNA nanotubes: (g) HR-TEM image of an unstained DNA nanotube (scale bar, 500 nm). (h) Zoom-in HR-TEM images of DNA nanotubes, exhibiting the cavities at the edges of the tubes (scale bar, 60 nm). (i) HR-TEM image of an uranyl-stained DNA nanotube (scale bar, 40 nm). Figure 3b,c shows numerous single-DNA nanotubes. It should be noted that the Figure 3b, showing numerous DNA nanotubes, is an exceptionally recorded image that presumably originated from the drying procedure. It is provided only to demonstrate the high yield of generated nanotubes. In fact, over 85% of the tubes are perfectly single nanotubes, such as depicted in Figure 3d and Supplementary Figure S1 (note that the histograms shown in Supplementary Fig. S2 are based on the analysis of only different single nanotubes). Furthermore, we find that the diameter of the resulting nanotubes is quite monodisperse and 74% of the resulting nanotubes exhibit a diameter of 60±5 nm. The SEM, AFM and transmission electron microscopy (TEM) images of typical single-DNA nanotubes are shown in Figure 3b–i and Supplementary Figure S1 . The length corresponds to 1.5–4 μm, the value of the synthesized RCA products ( Supplementary Fig. S3 ). Figure 3e depicts the SEM image of the edges of the nanotubes that clearly indicate the formation of the cavity in the tubes. Figure 3f depicts an AFM image of the resulting DNA nanostructures. Figure 3g,h depicts the TEM images of the unstained DNA nanotubes. Figure 3i shows the TEM image of the uranyl-stained DNA nanotubes. Periodical lines consisting of dark dots (corresponding to the cavities of the hexagons) are observed. The separation between the cavities is ca 10 nm, in agreement with the geometrical constrains. It should be noted that the length of the resulting nanotubes was confined by the heterogeneity of the RCA products ( Supplementary Fig. S3 ). In a control experiment the possible formation of nanotubes using a nucleic acid strand that included a non-complementary domain (VI′) to the sequence (III), was examined in the presence of the RCA template. No formation of DNA nanotubes or any other structures was observed. Figure 3: Self-assembly and images of single-DNA nanotubes comprised of hexagon subunits. ( a ) Schematic formation of a single-DNA nanotube through the self-assembly of the nucleic acid 'hexagon' subunit ( 1 ), in the presence of an RCA template ( 7 ) that is partially complementary to the hexagon subunits. ( b – e ) HR-SEM images of the resulting single-DNA nanotubes: ( b ) a collection of numerous nanotubes (scale bar, 2 μm). ( c ) Zoom-in image of the resulting nanotubes (scale bar, 150 nm). ( d ) A representative image of a single micrometre-long DNA nanotube (scale bar, 500 nm). ( e ) Zoom-in image of the edge of a single nanotube, exhibiting the cavity of the tube (scale bar, 300 nm). ( f ) AFM height image of a collection of separated DNA nanotubes (scale bar, 1.7 μm). ( g – i ) HR-TEM images of the DNA nanotubes: ( g ) HR-TEM image of an unstained DNA nanotube (scale bar, 500 nm). ( h ) Zoom-in HR-TEM images of DNA nanotubes, exhibiting the cavities at the edges of the tubes (scale bar, 60 nm). ( i ) HR-TEM image of an uranyl-stained DNA nanotube (scale bar, 40 nm). Full size image To further understand the mechanism of the formation of the DNA nanotubes, we designed a smaller nucleic acid hexagon subunit ( 4 ), that consists of 60 bases in the hexagon perimeter and a 10-base elongated toehold attached to the hexagon. The self-assembly of 4 , in the presence of the respective partially complementary RCA chain, led, similarly, only to single, non-branched DNA nanotubes, 80% of the nanotubes exhibit a diameter of 75±5 nm, ( Supplementary Figs S2 and S4 ). The study was further extended by examining the self-assembly of a nucleic acid strand ( 5 ), that can generate a tetragon-shaped subunit upon self-hybridization ( Fig. 4a ). The domains I and V are complementary to domain III, domain II is complementary to domain IV and domain VI acts as an auxiliary toehold for the secondary attachment of components. The self-assembly of single-stranded 'tetragons' ( 5 ) in the presence of the respective partially complementary RCA chain yielded, as before, only single-DNA nanotubes with lengths corresponding to the RCA chains. The diameter of the resulting nanotubes was, however, noticeably larger than that observed for the hexagon-type nanotubes. In all, 77% of the resulting nanotubes exhibit a diameter of 85±5 nm, see Supplementary Figure S2 . 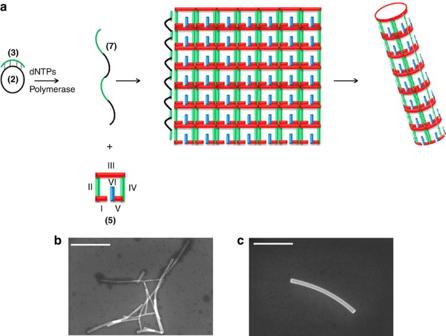Figure 4: Self-assembly and images of single-DNA nanotubes comprised of tetragon subunits. (a) Schematic formation of a single-stranded DNA nanotube through the self-assembly of a 'tetragon' nucleic acid subunit (5) in the presence of an RCA template (7) that is partially complementary to the 'tetragon' subunit. (b) HR-SEM image of a collection of DNA nanotubes consisting of 'tetragon' subunits (scale bar, 1 μm). (c) HR-SEM image of a representative DNA nanotube consisting of the 'tetragon' subunits (5) (scale bar, 500 nm). Figure 4: Self-assembly and images of single-DNA nanotubes comprised of tetragon subunits. ( a ) Schematic formation of a single-stranded DNA nanotube through the self-assembly of a 'tetragon' nucleic acid subunit ( 5 ) in the presence of an RCA template ( 7 ) that is partially complementary to the 'tetragon' subunit. ( b ) HR-SEM image of a collection of DNA nanotubes consisting of 'tetragon' subunits (scale bar, 1 μm). ( c ) HR-SEM image of a representative DNA nanotube consisting of the 'tetragon' subunits ( 5 ) (scale bar, 500 nm). Full size image The results reveal that the addition of the RCA blocker strand eliminated the bundling of the nanotubes, confined the lengths of the tubes to the dimensions of the RCA template, and that control over the diameter of the resulting nanotubes was achieved by the geometry of the self-organizing DNA subunits. We next formulated a model that may account for the unique features of the self-assembly of the single-DNA nanotubes. Formation of DNA nanotubes of controllable diameters Two different issues need to be addressed while suggesting a possible mechanism for the formation of these unique nanotubes: why does the RCA product induce the formation of single-DNA nanotubes and why are the resulting nanotubes of similar diameter, and how do the different subunits affect the resulting diameter? 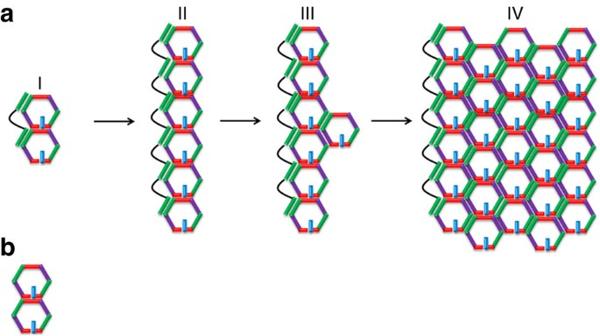Figure 5: Schematic mechanism for the dictated growth of non-branched DNA sheets consisting of the nucleic acid hexagon subunit (1). (a) Directional growth of the 'hexagon' subunits through the energetically favoured assembly of the subunits on the RCA template. (I) Initial assembly of two hexagon subunits and the RCA template that includes three hybridization domains. (II) The generation of a linear structure of hexagon subunits that includes three hybridization domains for each two neighbouring hexagon subunits and the RCA template. (III) Assembly of a new line of hexagon subunits. (IV) Assembly of a two-dimensional nanostructure. The nanostructure of the subunits with the DNA template acts as 'seed' for the directional growth of the sheet. (b) The energetically unfavoured 'seed' structure of two 'hexagons' that includes only one hybridization domain, before the growth of the sheet. Figure 5 depicts schematically the suggested mechanism for the favoured formation of the single nanotubes. We suggest that the RCA product introduces a 'seeding' mechanism for the formation of the 'graphene'-type hexagon sheet. In Figure 5a , the primary formation of the 'graphene'-type seeding sub-layer of the units on the RCA product is compared with the hybridization of subunits in the absence of the RCA ( Fig. 5b ). Evidently, the initial coupling of two hexagon subunits on the RCA product includes three hybridization domains, whereas the dimerization of two subunits that lack the RCA product includes only one hybridization domain, thus leading to the thermodynamically favoured template of hexagons on the RCA product, step II in Figure 5a . The hybridization of any hexagon subunit on any site of the template of hexagons yields a centre for the effective binding of the second hexagon, through three hybridization domains, step III. Accordingly, the addition of one hexagon to the template favours the directed growth of the 'graphene'-type sheet. One should note, however, that upon polymerization of the hexagons, the upper and lower edges of the sheets include hybridization domains that could lead, upon growing, to branched nanotubes. This possibility is, however, eliminated because of the micrometre dimensions of the RCA product, that drives the unidirectional growth of the array of subunits, compared with the nanometre dimensions of the edges, a feature that within the frame of the RCA template statistically favour the growth of the sheet. Figure 5: Schematic mechanism for the dictated growth of non-branched DNA sheets consisting of the nucleic acid hexagon subunit ( 1 ). ( a ) Directional growth of the 'hexagon' subunits through the energetically favoured assembly of the subunits on the RCA template. (I) Initial assembly of two hexagon subunits and the RCA template that includes three hybridization domains. (II) The generation of a linear structure of hexagon subunits that includes three hybridization domains for each two neighbouring hexagon subunits and the RCA template. (III) Assembly of a new line of hexagon subunits. (IV) Assembly of a two-dimensional nanostructure. The nanostructure of the subunits with the DNA template acts as 'seed' for the directional growth of the sheet. ( b ) The energetically unfavoured 'seed' structure of two 'hexagons' that includes only one hybridization domain, before the growth of the sheet. Full size image The control over the tube diameters by the geometry of the subunits and their mesh size can be accounted for using a plausible simple thermodynamic model (see Methods). According to this model, the thermodynamic stability of the tubes compared with the open sheets is dominated by two primary free energy contributions. The first is represented by the cohesion energy of the double-stranded DNA formed upon folding the sheet to a tube, the displacement of the RCA strand, and the adhering of the edges of the sheets through hybridization. (Note that the folding results in complete hybridization of the edges, whereas only partial hybridization of the edges with the RCA strand takes place). The cohesion energy depends on the length of binding of the DNA edges, their base sequence, and solution conditions such as salt concentration. Assuming that the cohesion energy per unit length of the tube along the nanosheet rim is ɛ , and that the length of the tube is l , the free energy gain upon the sheet adhering is given by F bind =− ɛl . The second free energy contribution is the elastic energy associated with the bending of the flat nanosheet into a tube. The nanosheet-bending energy is expected to be a function of the rigidity of the double-stranded DNA, which depends on the DNA persistence length, l p , the mesh geometry and the direction (axis) of the sheet folding. For a nanosheet with a bending modulus (in analogy to a spring constant), κ , the elastic energy associated with deforming the sheet into a tube of length l and radius R can be expressed using the Canham–Helfrich–Evans formalism [25] , [26] , [27] , [28] , where F bending = πlκ / R . Considering these two primary contributions to the free energy of tube formation from the nanosheet, F = F binding +F bending , we find that only above a threshold radius R* ∼ κ / ɛ , the free energy gain from binding compensates for the bending energy, thus thermodynamically favouring tube formation. For R < R* , the elastic energy for bending is larger than the binding energy, and hence, tube formation is disfavoured. For R > R* , the binding free energy gain, involved in the formation of the tubes, can compensate for the bending energy, and tube formation is favoured. Assuming that the sheet growth is slow (reversible), beyond a sheet width of 2 πR* (or slightly under due to thermal fluctuations) the sheet edges hybridize and form the tubes. The binding energy of duplex DNA is dominated by the base sequence and the length of the duplex, and was previously quantitatively estimated [29] . Similarly, bending energies of the different geometries of subunits and the free energy changes upon the respective base pairing can be quantitatively determined [30] , [31] , [32] . This enabled us to provide numerical estimates of κ and ɛ for the different nanosheet mesh geometries and the evaluation of the threshold R* values of the resulting nanotubes for the different geometries of the constituting subunits (for details of calculations and derived numerical values of κ , ɛ , and R* see Methods and Supplementary Information). Although the model relies on two approximately derived parameters, we find that with no adjustable parameters, the calculated dimensions of the resulting DNA nanotubes follow well the experimental results; R* large hexagons ≈30 nm, R* small hexagons ≈40 nm and R* tetragons ≈45 nm, leading to calculated diameters of 60 nm (experimental 60 nm), 80 nm (experimental 75) and 90 nm (experimental 85 nm) for the respective DNA nanotubes. Further applications of the resulting DNA nanotubes rest on the possibility to tether chemical components on the nanotubes' walls or to encapsulate materials in the tubes. The ordered organization of Au nanoparticles (NPs) tethered to the subunits of the DNA nanotubes was then examined ( Fig. 6 ). 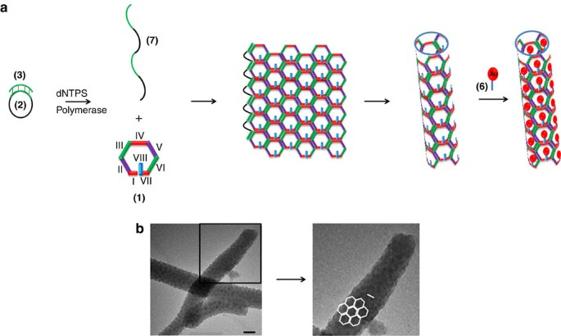Figure 6: Single-DNA nanotubes decorated with AuNPs. (a) The self-assembly of single-DNA nanotubes consisting of the 'hexagon' subunits (1) and tethered Au NPs (1.4 nm) to the 'hexagon' subunits. (b) HR-TEM images of the 'honeycomb' nanostructures consisting of the Au NPs tethered to the DNA nanotubes. Note that each of the hexagon subunits is decorated with an Au NP (scale bar left image, 20 nm; scale bar right image, 10 nm). The hexagon subunits in Figure 6a include a single-stranded nucleic acid chain that does not participate in the formation of the nanostructures, yet it provides an anchor to hybridize Au NPs (1.4 nm), functionalized with the nucleic acid, ( 6 ), that is complementary to the tethering units (VIII in 1 , 4 and VI in 5 ). Figure 6b depicts the HR-TEM image of the Au NPs attached to the hexagon-based nanotubes. A 'honeycomb' nanostructure showing the individual NPs in the respective hexagon is observed. The distance between adjacent NPs is ∼ 10 nm, in good agreement with the geometrical distance separating the centres of two adjacent hexagons. (Similarly, the ordered positioning of the Au NPs was achieved on the tetragon-based DNA nanotubes, Supplementary Fig. S5. ) Figure 6: Single-DNA nanotubes decorated with AuNPs. ( a ) The self-assembly of single-DNA nanotubes consisting of the 'hexagon' subunits ( 1 ) and tethered Au NPs (1.4 nm) to the 'hexagon' subunits. ( b ) HR-TEM images of the 'honeycomb' nanostructures consisting of the Au NPs tethered to the DNA nanotubes. Note that each of the hexagon subunits is decorated with an Au NP (scale bar left image, 20 nm; scale bar right image, 10 nm). Full size image This study introduces a paradigm to synthesize single-DNA nanotubes with controlled diameters. The method is based on the use of single-stranded nucleic acids that self-organize and oligomerize, because of complementary base pairing, into two-dimensional sheets of geometrically defined subunits that wrap into DNA nanotubes. The use of an RCA nucleic acid chain as a template for the directed growth of the two-dimensional sheet, and its functions in dictating the diameter of the resulting nanotubes were discussed. The physical model providing the relation between the geometry of the subunits and the resulting diameter of the nanotubes opens new dimensions in DNA nanotechnology. For example, by altering the hybridization energy of the base pairs comprising the subunits, for example, different bases or DNA/PNA pairs, further control over the diameters of the tubes may be achieved. Similarly, using other geometrical nucleic acid subunits, or mixing different geometrical structures, for example, octagon or hexagon/triangle mixture, may lead to nanotubes of other dimensions. Also, the tethering of other components to the nanotubes may yield new functionalities of these nanostructures. For example, linking cell-penetrating peptides to the nanotubes may provide new possibilities to trap chemical components in the nanotubes and guide them into cells. Theoretical model We describe here a simple model for the formation of simple DNA nanotubes by the assembly of geometrically confined nucleic acid subunits. By considering a simple free energy for nanotube formation, the model can be used to predict the radius of the resulting tubes. Details of the numerical estimates for parameters in the theoretical model are discussed in the Supplementary Information . Free energy of tube formation Let us consider a length l of DNA sheet ( Fig. 7 ) and calculate the free energy difference F associated with forming a tube from the sheet. We assume that this free energy contains only contributions from the cost of bending the sheet away from its flat configuration, and from a binding (cohesive) energy gain from the displacement of the RCA strand and formation of additional DNA base pairing contacts between single strands along the two sheet edges. All other contributions to the free energy are neglected. The free energy for the whole sheet in the tube configuration relative to the flat one is thus F = F el + F b , where F el is the elastic penalty to bending, and F b is the cohesive energy gain. 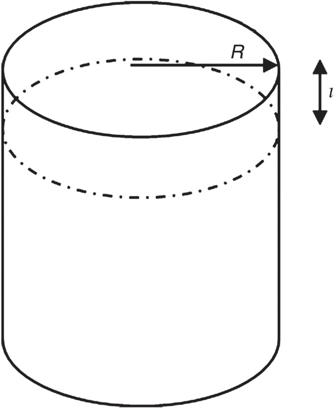Figure 7: Schematic of double-stranded DNA mesh closed into a tube. Relevant model parameters R and l are indicated. Figure 7: Schematic of double-stranded DNA mesh closed into a tube. Relevant model parameters R and l are indicated. Full size image The simplest model for the cylindrical bending deformation of a thin sheet is the Canham–Helfrich–Evans bending energy [26] , [27] , [28] , equation 1, where R is the sheet's radius of curvature (in this case—the radius of the cylindrical tube), κ is the bending modulus of the cylinder and R 0 is the spontaneous radius of curvature of the sheet. We shall assume here for simplicity that the spontaneous curvature of the sheet is zero, c 0 =1/ R 0 =0. The binding energy for the sheet linearly depends on the length of cylinder, where we have set ɛ as the (net) cohesive free energy per unit length. We note that this contribution may have entropic as well as energetic (enthalpic) contributions. The total free energy of the cylinder per unit length along the cylinder is given by equation 3, Clearly, this expression is only at a minimum for infinitely large closed sheets ( R →∞) that have no bending cost, but gain from cohesion. However, already beyond a certain radius of curvature R *= πκ / ɛ there is a net free energy gain for forming a tube. If the growth of the sheet is very slow (reversible) so that the sheet's free ends have time to find each other and bind, then beyond a sheet width of 2 πR * the sheet would close to form a tube. In reality, however, the sheet is continuously growing, so that a competition develops between sheet widening and tube closing. This is expected to result in a distribution of sizes starting at R * (or slightly before, because of thermal fluctuations) and beyond. Once a sheet closes on itself into a tube, kinetics can be assumed to arrest, because of the high barriers associated with opening a tube once it is closed. We note that our approach is somewhat analogous to the determination of the size of lipid vesicles formed from open edged membrane sheets that derives from a similar competition between elastic and edge energies [33] . The main result of this highly simplified model is that the tube radius scales as R * ∼ κ / ɛ . Namely, the more it costs to bend, the larger the radius, whereas the larger the cohesion gain for closing a tube, the smaller the radius. A tendency to form the smallest tubes possible (once the formation free energy is negative) can be explained by the entropic requirement for maximal number of particles (tubes) in solution. Interestingly, this kind of requirement is also recognized as an important consideration in the formation of spherical micelles rather than other larger aggregates in surfactant solutions. Conversely, entropy due to sheet undulations in the open form should disfavour tube closure, but this latter contribution is probably small for the rather stiff nanosheets considered here. Materials Oligonucleotides and chemicals were purchased from Sigma-Genosys, unless noted otherwise. Microspin G-25 (Sephadex) columns were purchased from Illustra. Ultrapure water from a NANOpure Diamond (Barnstead source was used throughout all the experiments). Quick ligation kit and Phi29 DNA polymerase were purchased from New England Biolabs. Mono-sulfo- N -hydroxysuccinimide Au NPs were purchased from Nanoprobes. Microcon filtration devices were purchased from Millipore. General methods Atomic force microscopy (AFM) imaging was performed at room temperature using a multimode scanning probe microscope with a Nanoscope 3A controller (Digital Instruments/Veeco Probes). AFM images were recorded on samples of 10 μl of DNA self-assembled nanostructures, deposited on freshly cleaved mica surfaces (Structure Probe, Inc.), and dried in a chemical hood. Images were taken with NSC 15 AFM tips (Mikromasch) using the tapping mode at their resonant frequency. The images were analysed with WsXM SPIP software (Nanotec, Inc.). SEM images were taken with a Sirion HR-SEM on silicon slides (Virginia semiconductor, Inc.), slides were first washed with distilled water followed by ethanol and acetone wash, then UV/ozone cleaned using a T1O×10/OES/E UV/ozone chamber from UVOCS, Inc., followed by treatment of the surface with 2% aminopropyltriethoxysilane for 30 min, and heated to 110 °C for 10 min to generate an amino monolayer. HR-TEM images of the Au NP-labelled nanotubes were taken with a HR-TEM Tecnai F-20 G 2 and performed on copper/formvar/carbon 400 mesh grids from Electron Microscopy Sciences. For negatively stained samples, 5 μl of the sample solution was adsorbed for 2 min, then a 2% uranyl acetate solution was added for 2 min, washed with double-distilled water and gently dried. The unstained images were collected on a Zeiss Libra 200MC machine operated at an accelerating voltage of 200 kV. Oligonucleotides: 1 5′-TTATTATTATACATACATACATATTAGTTAGTTAGTTAAATAATAATAATAATTATGTATGTATGTATTAACTAACTAACTAAATTATTAGACGACGACG-3′ 2 5′-ATACATACATACATAAAAAAAAAAAAAAAA-3′ or for the short hexagon: 5′-ATACATACATAAAAAAAAAA-3′ 3 5′-TATGTATTTTTTTTT-3′ 4 5′-TTATTATACATACATTTAGTTAGTTAATAATAATAATGTATGTATAACTAACTAATATTAGACGACGACG-3′ 5 5′-ATACATACATACATATTAGTTAGTTAGTTATATGTATGTATGTATTAACTAACTAACTAAGACGACGACG-3′ 6 5′-CGTCGTCGTC-3′ Preparation of DNA nanostructures Oligonucleotides: ( 1 ) 5′-TTATTATTATACATACATACATATTAGTTAGTTAGTTAAATAATAATAATAATTATGTATGTATGTATTAACTAACTAACTAAATTATTAGACGACGACG-3′ or ( 4 ) 5′-TTATTATACATACATTTAGTTAGTTAATAATAATAATGTATGTATAACTAACTAATATTAGACGACGACG-3′ or ( 5 ) 5′-ATACATACATACATATTAGTTAGTTAGTTATATGTATGTATGTATTAACTAACTAACTAAGACGACGACG-3′ were mixed in a phosphate buffer solution 1×10 −4 litre (1×10 −5 M, pH 7.4), in a final concentration of 1×10 −7 M, heated to 94 °C for 10 min, and then cooled down to room temperature (25 °C) at a rate of 1 °C per 15 min. Preparation of rolling circle amplification DNA products Oligonucleotides: ( 2 ) 5′-ATACATACATACATAAAAAAAAAAAAAAAA-3′ or 5′-ATACATACATAAAAAAAAAA-3′ 1×10 −6 M were ligated following a quick ligation protocol (NEB) using the oligonucleotide ( 3 ) 5′-TATGTATTTTTTTTT-3′ 1×10 −5 M as the RCA primer to form a ligated circular DNA, in quick ligation buffer, 5×10 −5 litre. Then, 2.5×10 −6 litre of the ligated circular oligonucleotide was treated with 0.5×10 −3 M dNTPs, and 0.8 U of Phi29 DNA polymerase in 5×10 −5 litre of Phi29 buffer for 1 h, at 30 °C, the enzymes were then deactivated at 65 °C for 10 min. A volume of 2×10 −6 litre of the RCA product was then added to 1×10 −7 M of the hexagon/tetragon oligonucleotides in phosphate buffer solution 1×10 −4 litre (1×10 −5 M, pH 7.4), heated to 94 °C for 10 min, and then cooled down to room temperature (25 °C) at a rate of 1 °C per 15 min. Preparation of ( 6 )-modified Au NPs A concentration of 5×10 −6 M of the amino-modified oligonucleotide ( 6 ) 5′-CGTCGTCGTC-3′ was mixed with 5×10 −5 M of N -hydroxysuccinimide active ester modified 1.4 nm. Au NPs (Nanoprobes) in a phosphate buffer solution (1×10 −2 M, pH 7.4) 1×10 −4 litre, for 40 min, and then the excess Au NPs were separated using microspin G-25 (sephadex) columns. Then, 5×10 −6 litre of 6 -modified Au NPs was hybridized with the nanostructures generated by ( 1 ), ( 4 ) or ( 5 ) that were hybridized with the RCA product, 2.5×10 −5 litre, in phosphate buffer solution 5×10 −5 litre (1×10 −5 M, pH 7.4) for 30 min at room temperature. Samples were then purified using a 100,000 Microcon device (Millipore) following the manufacturer's protocol. How to cite this article: Wilner, O. I. et al . Self-assembly of DNA nanotubes with controllable diameters. Nat. Commun. 2:540 doi: 10.1038/ncomms1535 (2011).